Supramolecular high-aspect ratio assemblies with strong antifungal activity Efficient and pathogen-specific antifungal agents are required to mitigate drug resistance problems. Here we present cationic small molecules that exhibit excellent microbial selectivity with minimal host toxicity. Unlike typical cationic polymers possessing molecular weight distributions, these compounds have an absolute molecular weight aiding in isolation and characterization. However, their specific molecular recognition motif (terephthalamide-bisurea) facilitates spontaneous supramolecular self-assembly manifesting in several polymer-like properties. Computational modelling of the terephthalamide-bisurea structures predicts zig-zag or bent arrangements where distal benzyl urea groups stabilize the high-aspect ratio aqueous supramolecular assemblies. These nanostructures are confirmed by transmission electron microscopy and atomic force microscopy. Antifungal activity against drug-sensitive and drug-resistant strains with in vitro and in vivo biocompatibility is observed. Additionally, despite repeated sub-lethal exposures, drug resistance is not induced. Comparison with clinically used amphotericin B shows similar antifungal behaviour without any significant toxicity in a C. albicans biofilm-induced mouse keratitis model. The number of opportunistic fungal infection cases is increasing due to growing populations of immunocompromised patients [1] . These invasive infections are mainly caused by Candida and Asper g illus species as well as Cryptococcus neoformans ( C. neoformans ). It has been reported that candidiasis, a fungal infection caused by Candida , was the third most common blood stream infection in the United States [2] , [3] . Fungal infections resistant to conventional antifungal drugs have been increasingly documented [4] , [5] , and many existing antifungal agents (for example, triazoles and polyenes) have witnessed resistance development in patients [1] . This is of huge concern within health-care and clinical settings due to the extremely limited selection of antifungal agents. Another challenge in developing antifungal drugs is that fungi are metabolically similar to mammalian cells, providing limited fungi-specific targets. For example, amphotericin B has broad-spectrum antimicrobial activities by binding ergosterol, the key sterol in fungal membrane, to form aggregates [6] . These aggregates induce membrane pores resulting in cell lysis. In a similar fashion, amphotericin B can also bind cholesterol in mammalian cell membranes, leading to non-specific toxicity. Haemolysis and nephrotoxicity are commonly reported side-effects caused by this drug in patients [7] . In aggregate, all these issues have created a pressing need for the development of novel antifungal agents that are efficient and pathogen-specific. Host defence peptides and synthetic polymers are two classes of macromolecules currently being studied as effective antimicrobials [8] , [9] , [10] , [11] . These materials are amphiphilic while also carrying cationic charge. They selectively interact and disintegrate negatively charged microbial walls or membranes via electrostatic interactions and insertion into membrane lipid domains. In addition, it is difficult for microbial cells to repair a physically damaged cell wall or membrane, hence avoiding potential microbial resistance development. Despite their efficacious antimicrobial activity, both peptides and synthetic polymers have seen limited clinical applications because of several inherent problems. For example, antimicrobial peptides generally have a short half-life in vivo due to enzymatic degradation, and suffer from high production costs. Bio-inspired synthetic polymers have been reported and have achieved considerable success in overcoming some of the drawbacks found with antimicrobial peptides, but many of them are cytotoxic to mammalian cells. In this study, we describe the synthesis, self-assembly and therapeutic activity for a novel class of discrete low-molecular weight antifungal agents. Their chemical structures are designed to incorporate specific molecular recognition motifs that induce formation of high-aspect ratio supramolecular assemblies. The assembled structures have polymer-like properties including a glass transition temperature ( T g ), and fibre-like morphologies in water. Compared with discrete molecules, fibre formation increases local concentration of cationic charges and compound mass, which facilitates the targeting and subsequent fungal membrane lysis with high efficiency and minimal haemolysis/cytotoxicity at concentrations far exceeding the therapeutic dosage. The nano-assemblies are effective against clinically isolated drug-resistant fungi and fungal biofilm, and prevent drug resistance development. In a fungal keratitis mouse model, these nanostructures decrease the severity of keratitis without causing any toxicity. Compound synthesis and characterization A key design motif of these small molecules was the rigid terephthalamide diamine that was readily modified to generate cationic terephthalamide-bisurea amphipathic compounds. These monodisperse molecules were constructed in a one-pot synthesis by reaction of a diamine with bis(pentafluorophenyl)carbonate generating reactive carbamates ( Fig. 1 ). Subsequent reaction with an alkyl diamine, where a single amine group was previously protected by tert -butyloxycarbonyl ( t Boc), generated the terephthalamide-bisurea compound readily isolated by precipitation into ether. These compounds were then dissolved in trifluoroacetic acid (TFA) (20 h) for removal of t Boc groups and generation of amine/TFA salts, again isolated by simple precipitation in ether. Four compounds were prepared having ethyl, butyl, hexyl and benzyl amine spacers between the urea and cationic charge, with absolute molecular weights ranging from 774.7 to 926.9 g mol −1 ( Supplementary Figs S1–S4 ; Supplementary Table S1 and Supplementary Methods ). 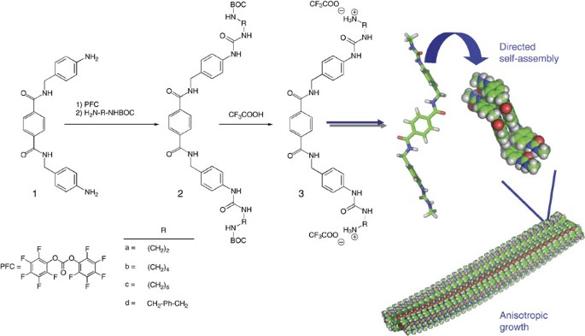Figure 1: Synthesis and characteristics of compounds 3a–d. Self-assembly motif with tunable functional groups. Molecular mechanics conformational analysis of the terephthalamide-bisurea structure revealed a zig-zag or bent structure with the distal benzyl urea groups perpendicular to the terephthalamide nanorod structure that is mechanically stable and is capable of generating high aspect structures. Figure 1: Synthesis and characteristics of compounds 3a–d. Self-assembly motif with tunable functional groups. Molecular mechanics conformational analysis of the terephthalamide-bisurea structure revealed a zig-zag or bent structure with the distal benzyl urea groups perpendicular to the terephthalamide nanorod structure that is mechanically stable and is capable of generating high aspect structures. Full size image Interestingly, these compounds did not show a melting point, but rather manifested a T g as confirmed by both differential scanning calorimetry (DSC) and dynamic mechanical analysis (DMA) performed on a solid support. For example, compound 3b showed a T g at ~120 °C (DSC), and an associated modulus drop and tan δ increase via DMA ( Fig. 2a,b ). These findings indicated similarities to the amorphous glasses synthesized by Ober et al. [12] , low molecular weight resist compounds that have a T g , low viscosity and distinctive dissolution properties due to the lack of molecular weight distribution. Furthermore, the aforementioned compounds formed supramolecular structures with cationic surfaces (zeta potential: 32–45 mV) when dissolved in water above their critical micellar concentrations (CMCs) (12-100 mg l −1 in de-ionized water; 6–56 mg l −1 in the fungus culture medium) ( Table 1 ). For example, 3b and 3d formed the nanofibers (several μm and several hundred nm in length, ~5 nm and ~10 nm in diameter, respectively) after dialysis against water, as seen by transmission electron microscopy (TEM) ( Fig. 2d,e , respectively). Interestingly, 3b self-assembled into nanofibers with high flexibility, while 3d formed relatively rigid nanofibers presumably due to its rigid molecular structure. Solution atomic force microscopy (AFM) of 3b ( Fig. 2c ) also shows anisotropic structures, although of considerably shorter lengths. Molecular mechanics conformational analysis of the terephthalamide-bisurea core structure revealed a zig-zag or bent structure with distal benzyl urea groups perpendicular to the terephthalamide core ( Fig. 1 and Supplementary Fig. S5 ). These zig-zag structures pack together into planar sheets stabilized by urea–urea hydrogen bonds and aromatic stacking. As the amide and urea groups are perpendicular, planar sheets further stack against one another, stabilized by hydrophobic interactions and amide–amide hydrogen bonds, generating a multilayer nanorod ( Fig. 1 and Supplementary Fig. S5 ). This cross-braced nanorod structure is mechanically stable and allows high-aspect ratio structures. 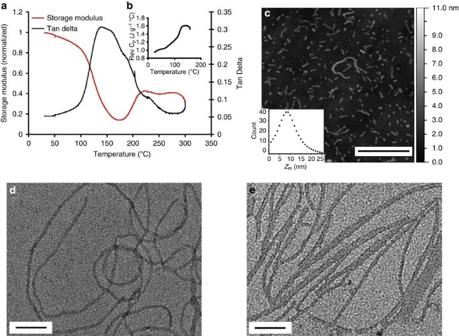Figure 2: Polymer-like properties. (a) DMA and (b) DSC thermograms of compound3a. (c) Topography micrograph of supramolecular assemblies of3busing AFM in fluid. Sample was prepared by direct dissolution of compound3bin water and imaged under water. The inset shows a distribution of statistical mean height (zm) obtained through particle analysis. A Lorentzian fit to the distribution gives azmof ~8 nm in water. Scale bar: 500 nm. TEM micrographs of (d) compound3band (e) compound3d. Scale bar: 100 nm. Figure 2: Polymer-like properties. ( a ) DMA and ( b ) DSC thermograms of compound 3a . ( c ) Topography micrograph of supramolecular assemblies of 3b using AFM in fluid. Sample was prepared by direct dissolution of compound 3b in water and imaged under water. The inset shows a distribution of statistical mean height ( z m ) obtained through particle analysis. A Lorentzian fit to the distribution gives a z m of ~8 nm in water. Scale bar: 500 nm. TEM micrographs of ( d ) compound 3b and ( e ) compound 3d . Scale bar: 100 nm. Full size image Table 1 Physicochemical and biological properties of the cationic compounds. Full size table In vitro antifungal activity We evaluated these cationic assemblies for antifungal activity against clinically relevant C. albicans , clinically isolated drug-sensitive and drug-resistant C. neoformans fungi. The overall net cationic charge of the assemblies allowed sufficient electrostatic interactions with anionic fungal cell surfaces. The compounds 3a – 3d inhibited fungal growth at relatively low minimum inhibitory concentration (MIC) values, which were greater than their CMCs in the fungus culture medium ( Table 1 ). In addition, MIC values remained unchanged when the fungal concentration varied from 10 2 to 10 5 CFU ml −1 ( Supplementary Fig. S6 ). These findings indicated that the compounds were active as aggregate assemblies rather than discrete molecules. This is particularly important as the cell wall of C. albicans consists of multiple layers with low negative charges (zeta potential: −4 mV), which impairs the ability of cationic nanoparticles to adhere to the cell wall and cause membrane disruption and lysis. The antifungal activity might be attributed to the nanostructure formation ( Fig. 2c ), facilitating cell wall/membrane penetration. Additionally, increasing hydrophobicity of the terminal groups from (CH 2 ) 2 ( 3a ) to (CH 2 ) 4 ( 3b ) improved antifungal efficacy ( Fig. 1 ). However, further increasing the hydrophobicity from (CH 2 ) 4 to (CH 2 ) 6 ( 3c ) did not affect antifungal activity. The compound 3d that can form rigid nanofibers had higher efficacy against C. neoformans as compared with 3a – 3c . In order to determine microbicidal properties, colony assays were performed. Fluconazole demonstrated fungistatic characteristic against C. albicans (MIC: 2 mg l −1 ) ( Fig. 3a ) and C. neoformans (MIC: 8 mg l −1 ) ( Fig. 3b ) even at 2 × MIC. At these concentrations, the reduction in the viable colony counts of fungi after treatment with fluconazole was <3 log 10 as compared with the control without the treatment. This phenomenon was also reported by others [13] . However, C. albicans and C. neoformans treated with the assemblies for 24 h showed >3 log 10 reduction in the viable colony counts as compared with the control group (that is, >99.9% eradication) using concentrations at their MIC ( Fig. 3a,b ), and they were almost completely killed (~100%) at 2 × MIC, indicating a fungicidal mechanism. The capability of cationic compounds for killing fungi was further investigated by analysing the viable colony counts of C. albicans upon treatment at MIC concentration utilizing various exposure times. Notably, >80% of C. albicans cells exposed to 3b were killed at 30 min, and >99.9% eradication was found at 1 h ( Supplementary Fig. S7 ). 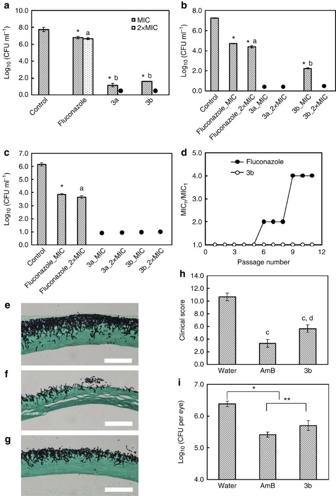Figure 3:In vitroandin vivoantifungal activity. Viable colony counts (Log10) of (a)C. albicansand (b)C. neoformansafter being treated with3a,3band fluconazole at the specified concentrations for 24 h. (c) Viable colony counts (Log10) ofC. neoformans(clinically isolated fluconazole-resistant strain) after treatment with3aor3bat the specified concentrations for 24 h; fluconazole was used as the control. *P<0.01,3a,3band fluconazole at their respective MICs versus control;a:P>0.05, fluconazole at 2 × MIC versus fluconazole at MIC;b:P<0.001,3a,3bat MIC versus fluconazole at MIC. Filled black circles indicate that no colony was observed. (d) Changes in MICs of antifungal agents upon multiple sub-lethal exposures. (e–g) Representative histological sections of mouse cornea treated with water (e), AmB (f) and3b(g) (Grocott’s methenamine silver stain, fungi in black). Scale bar: 100 μm. (h) Clinical scores for keratitis after treatment with the topical eye drop solutions. A total score of ≤5, 6–9 and >9 indicate mild, moderate and severe keratitis, respectively.c:P<0.0005,3band AmB versus control;d:P=0.008,3bversus AmB. (i) CFU ofC. albicansin mouse cornea treated with AmB and3b. The data are expressed as mean±s.d. of 3–6 replicates. *P<0.01,3band AmB versus control. **P>0.05,3bversus AmB. Figure 3: In vitro and in vivo antifungal activity. Viable colony counts (Log 10 ) of ( a ) C. albicans and ( b ) C. neoformans after being treated with 3a , 3b and fluconazole at the specified concentrations for 24 h. ( c ) Viable colony counts (Log 10 ) of C. neoformans (clinically isolated fluconazole-resistant strain) after treatment with 3a or 3b at the specified concentrations for 24 h; fluconazole was used as the control. * P <0.01, 3a , 3b and fluconazole at their respective MICs versus control; a : P >0.05, fluconazole at 2 × MIC versus fluconazole at MIC; b : P <0.001, 3a , 3b at MIC versus fluconazole at MIC. Filled black circles indicate that no colony was observed. ( d ) Changes in MICs of antifungal agents upon multiple sub-lethal exposures. ( e – g ) Representative histological sections of mouse cornea treated with water ( e ), AmB ( f ) and 3b ( g ) (Grocott’s methenamine silver stain, fungi in black). Scale bar: 100 μm. ( h ) Clinical scores for keratitis after treatment with the topical eye drop solutions. A total score of ≤5, 6–9 and >9 indicate mild, moderate and severe keratitis, respectively. c : P <0.0005, 3b and AmB versus control; d : P =0.008, 3b versus AmB. ( i ) CFU of C. albicans in mouse cornea treated with AmB and 3b . The data are expressed as mean±s.d. of 3–6 replicates. * P <0.01, 3b and AmB versus control. ** P >0.05, 3b versus AmB. Full size image The antifungal effect of 3a and 3b was further investigated against clinically isolated fluconazole-resistant C. neoformans . MIC of fluconazole against this strain of fungus increased from 2 (against drug-sensitive strain) to 62.5 mg l −1 , verifying that this strain of fungus was resistant to fluconazole [14] . The MICs of 3a and 3b were 125.0 and 62.5 mg l −1 , respectively, which were the same as those against drug-sensitive C. neoformans . At and above their MICs, both cationic assemblies removed almost 100% fluconazole-resistant C. neoformans cells, while fluconazole was fungistatic as expected (reduction in the viable colony counts of fungi after fluconazole treatment: <3 log 10 as compared with the control without the treatment) ( Fig. 3c ). These results indicated that 3a and 3b were effective against both drug-sensitive and drug-resistant fungi. Furthermore, multiple sub-lethal dose treatments of C. albicans with cationic assemblies did not induce resistance. In contrast, drug resistance was developed after six sub-lethal fluconazole exposures ( Fig. 3d ). In addition, the cationic assemblies were fungicidal at MIC with >99.9% killing efficiency of C. albicans at passages 1–11, while fluconazole was fungistatic towards C. albicans even at 62.5 × MICs ( Supplementary Fig. S8 ). These findings demonstrated great potential of the cationic assemblies against drug resistance. Biofilm lysis Medical implants beset by fungal biofilm formations, especially those that are resistant to clinical antifungal agents such as amphotericin B and fluconazole [15] , [16] , are a major cause for device failures. To evaluate biofilm disruption ability, cationic assembly 3b was utilized for the treatment of contact lenses having a C. albicans biofilm in order to mimic fungal keratitis in vitro [17] . The untreated biofilm consisted of both metabolically active oval and long tubular hyphae cell types (red region), where extracellular matrix (ECM) (green region) was bound in both of them ( Fig. 4a,c ). In contrast, 3b treatment mediated a significant reduction in the metabolically active cells ( Fig. 4d ), and cell wall/membrane of C. albicans was broken and debris was observed after the treatment ( Fig. 4b ). XTT and Safranin assays further confirmed the drastic decrease in C. albicans survival and the biofilm disruption after 3b treatment ( Supplementary Fig. S9 ). 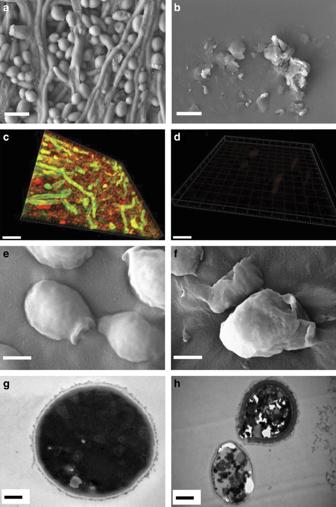Figure 4: Biofilm disruption and antifungal mechanism studies. SEM images ofC. albicansbiofilms (a) before and (b) after treatment with3b(scale bar: 5 μm). Confocal images ofC. albicansbiofilms (c) before and (d) after treatment with3b(scale bar: 20 μm). Areas of green fluorescence represents biofilm ECM stained with CON-A, and red fluorescence represents metabolically active cells stained with FUN-1. SEM images ofC. albicans(e) before and (f) after treatment with3b(scale bar: 1 μm). TEM images ofC. neoformans(g, scale bar: 0.5 μm) before and (h, scale bar: 1 μm) after treatment with3b. Figure 4: Biofilm disruption and antifungal mechanism studies. SEM images of C. albicans biofilms ( a ) before and ( b ) after treatment with 3b (scale bar: 5 μm). Confocal images of C. albicans biofilms ( c ) before and ( d ) after treatment with 3b (scale bar: 20 μm). Areas of green fluorescence represents biofilm ECM stained with CON-A, and red fluorescence represents metabolically active cells stained with FUN-1. SEM images of C. albicans ( e ) before and ( f ) after treatment with 3b (scale bar: 1 μm). TEM images of C. neoformans ( g , scale bar: 0.5 μm) before and ( h , scale bar: 1 μm) after treatment with 3b . Full size image Antifungal mechanism The antifungal mechanism was studied by visualizing a typical cell structure (that is C. neoformans and C. albicans ) before and after treatment via scanning electron microscopy (SEM) and TEM. Prior to treatment, all fungi showed smooth cellular exteriors and intact cell wall/membrane ( Fig. 4e,g —control). After treatment with 3b , cell wall and membrane damage was easily visible along with dead microbe remnants ( Fig. 4f,h —treated). In particular, the membrane damage led to the release of cytoplast from C. neoformans cells ( Fig. 4h ). Fungal membrane damage was also evaluated by measuring the absorbance (260 nm) of cell culture media, which can be directly correlated with nucleic acid release post-treatment [18] . As shown in Supplementary Fig. S10 , following treatment of C. albicans with 3b , a significant amount of nucleic acids was observed in the culture media. Furthermore, nucleic acid release was found to be dose-dependent with elevated concentrations of 3b , causing amplified membrane damage, thereby inducing more cytoplasmic leakage. We postulated that cationic nanorods exploited an associative mechanism (which required appropriately balanced hydrophobic and hydrophilic regions), whereby antifungal material became integrated within the cellular exterior causing membrane destabilization and lysis. This membrane-lytic antifungal mechanism might be the reason for preventing the development of drug resistance ( Fig. 3d ). In vitro biocompatibility A major side effect caused by many cationic antimicrobial peptides and polymers is haemolysis. Haemolytic evaluations were conducted using rat red blood cells incubated with the compounds at various concentrations ( Supplementary Fig. S11a ). Negligible haemolytic activity was observed for all samples, even at concentrations well above the MIC (up to 1,000 mg l −1 ), demonstrating excellent selectivity. To evaluate cytotoxicity towards mammalian cells, human dermal fibroblast viability was analysed via MTT assay after incubation with compounds at various concentrations (15.6–1,000 mg l −1 ) for 24 h ( Supplementary Fig. S11b ). More than 83% of cells were viable at all concentrations tested, indicating excellent mammalian cell biocompatibility. In vivo antifungal efficacy To evaluate the in vivo antifungal activity of cationic compounds, fungal keratitis was established in mice by using contact lens-associated C. albicans biofilm infection [19] , [20] . The experimental protocol was approved by the Institutional Animal Care and Use Committee of Biological Research Centre, Agency for Science, Technology and Research (A*STAR), Singapore. This disease model was chosen because fungal keratitis is a severe eye infection and a major cause of ocular morbidity. An eye ulcer with dense opaque appearance was seen on the eyeballs of the mice with keratitis. The mice were randomly grouped and treated with three topical eye drop solutions: water solution (control), 3b (2,000 mg l −1 ) and amphotericin B (AmB) (1,500 mg l −1 ). AmB was selected as positive control instead of fluconazole because AmB is a clinically used strong antifungal agent, while fluconazole was unable to clear C. albicans biofilm in vitro . In control animals receiving water as eye drops, histological analysis showed extensive hyphal invasion into the corneal stroma ( Fig. 3e ). In contrast, treatments with 3b and AmB resulted in significant reduction in the hyphal invasion ( Fig. 3f,g and Supplementary Fig. S12 ), although AmB was relatively more potent. The maximal depth of fungal invasion in the cornea treated with AmB and 3b was remarkably reduced as compared with that in the control group (18.0±2.1 and 27.6±1.5 μm versus 63.4±5.6 μm) ( Supplementary Fig. S12 ). Keratitis in the control, AmB- and 3b -treated groups was further evaluated to provide clinical scores of 10.7±0.6, 3.3±0.6 and 5.7±0.6, respectively ( Fig. 3h and Supplementary Fig. S13 ), demonstrating that AmB and 3b treatment significantly lessened the severity of keratitis ( P <0.0005). Importantly, 3b treatment reduced the number of viable fungi remaining on the eyeballs (measured in colony-forming unit (CFU)) (5.79 log 10 CFU per eye versus 6.38 log 10 CFU per eye for control, 74.3% reduction, P <0.01) as effectively as AmB (5.44 log 10 CFU per eye, 88.7% reduction, P >0.05 as compared with 3b treatment) ( Fig. 3i ). Moreover, no significant erosion was observed in the epithelium of mouse cornea after topical administration of 3b ( Supplementary Fig. S14 ), indicating that 3b was biocompatible to the corneal epithelium and underlying stroma. AmB has poor solubility in water and is unstable in aqueous, acidic or alkaline solution [21] . The water-soluble and stable antifungal compound 3b is a better alternative to AmB. As fungi are metabolically similar to mammalian cells, limited fungi-specific targets are available for host differentiation. There is a pressing need to develop efficient and pathogen-specific antifungal agents to mitigate growing drug resistance problems. Our results show that a novel class of pathogen-specific, low-molecular weight antifungal agents have been successfully synthesized for self-assembly and therapeutic activity. These compounds have an exact molecular weight with a specific molecular recognition motif imparting polymer-like solid state properties— T g and fibre-like assembly in water. The multivalent cationic charges of the self-assembled nanostructures facilitated lysis of fungal membranes with low MIC values and high selectivity. The cationic assemblies demonstrated efficient antifungal activity against clinically isolated drug-resistant strains, and effectively dispersed biofilms. In addition, they did not develop drug resistance after multiple sub-lethal treatments due to their membrane-lytic antifungal mechanism. Importantly, the nano-assemblies significantly decreased fungal counts, hindered hyphal corneal invasion and reduced the severity of keratitis in a fungal keratitis mouse model. They were also shown to have excellent in vitro and in vivo biocompatibility. Therefore, these small-molecule compounds hold great potential as antifungal agents for the prevention and treatment of topical fungus-induced infections where large and local doses can be administered. PET degradation with 4-aminobenzylamine PET flakes (9.61 g, 0.05 mol), 4-aminobenzylamine (28.2 g, 0.23 mol) and TBD (0.36 g, 2.5 mmol) were placed in a 250-ml flask, and then heated under nitrogen atmosphere at 120 °C for 3 h during which the reaction mixture solidified. The mixture was triturated and washed in isopropanol (200 ml). The residue was rinsed with THF and diethylether several times, and then dried in a vacuum oven at 80 °C, yielding a white powder as a product, bis(4-aminobenzyl)terephthalamide (4ABTA: 15.15 g, 81%). 1 H-NMR (400 MHz, dimethyl sulfoxide (DMSO)- d 6 ): δ 8.96 ( t , J =6 Hz, 2H, N H ), 7.93 ( s , 4H, Ar- H ), 6.98 ( d , J =8 Hz, 4H, Ar- H ), 6.51 ( d , J =8 Hz, Ar- H ), 4.96 ( s , 4H, N H 2 ), 4.30 ( d , J =6 Hz, 4H, C H 2 ). 13 C-NMR (100 MHz, DMSO- d 6 ): δ 165.4, 147.6, 136.7, 128.4, 127.3, 126.4, 113.8, 42.5. m.p. (DSC): 203 °C. The brief procedure for preparation of compound 3b is given below as a typical example. Synthesis of compound 3b To a dry dimethylformamide (DMF) solution (16 ml) of pentafluorophenyl carbonate (PFC) (3.97 g, 10.1 mmol) was added a dry DMF solution (8 ml) of the diamine, N 1 , N 4 -bis(4-aminobenzyl)terephthalamide (4ABTA, 1 ) (1.50 g, 4.0 mmol). The reaction mixture was stirred for 1 h at room temperature. Subsequently, tert -butyl (4-aminobutyl)carbamate (2.36 g, 12.6 mmol) was added, and the mixture was kept stirring overnight. To remove excess PFC and the amine reagent, the reaction mixture was precipitated in diethylether (250 ml). Thereafter, the product was filtered and dried in vacuum (60 °C) to yield 2b (2.87 g, 90%). 1 H-NMR (400 MHz, DMSO- d 6 ): δ 9.08 ( t , J =5.8 Hz, 2H, Ar-CON H ), 8.36 ( s , 2H, Ar-N H ), 7.95 ( s , 4H, Ar- H ), 7.32 ( d , J =8.4 Hz, 4H, Ar- H ), 7.17 ( d , J =8.4 Hz, 4H, Ar- H ), 6.82 ( t , J =5.6 Hz, 2H, N H COO), 6.07 ( t , J =5.6 Hz, 2H, N H CH 2 ), 4.39 ( d , J =5.6 Hz, 2H, Ar-C H 2 ), 3.09–3.00 ( m , 4H, C H 2 NHCOO), 2.95–2.86 ( m , 4H, NHC H 2 ), 1.41–1.32 ( m , 26H, C H 2 and C H 3 ). 13 C-NMR (100 MHz, DMSO- d 6 ): 165.3, 155.5, 155.1, 139.3, 136.6, 131.8, 127.7, 127.2, 117.4, 77.3, 42.2, 39.6, 38.7, 28.2, 27.2, 27.0. The compound 2b (2.50 g, 3.11 mmol) was added into trifluoroacetic acid (TFA, 10 ml) and the mixture was stirred overnight. As the deprotection proceeded, the reaction mixture became homogeneous. The reaction mixture was then precipitated in diethylether (200 ml), and the precipitate was filtered and washed with diethylether a few times, and dried in vacuum (60 °C) to yield 3b (2.07 g, 80%). 1 H-NMR (400 MHz, DMSO- d 6 ): δ 9.09 ( t , J =5.8 Hz, 2H, Ar-CON H ), 8.56 ( s , 2H, Ar-N H ), 7.95 ( s , 4H, Ar- H ), 7.72 ( b , 6H, N H 3 + ), 7.34 ( d , J =8.4 Hz, 4H, Ar- H ), 7.17 ( d , J =8.4 Hz, 4H, Ar- H ), 6.30 ( t , J =5.8 Hz, 2H, N H CH 2 ), 4.39 ( d , J =5.6 Hz, 2H, Ar-C H 2 ), 3.08 ( ddd , J =6.2, 6.2, 6.0 Hz, 4H, C H 2 NH), 2.80 ( t , J =7.4 Hz, 4H, C H 3 ), 1.59–1.39 ( m , 8H, C H 2 ). 13 C-NMR (100 MHz, DMSO- d 6 ): 165.3, 158.4, 155.3, 139.4, 136.6, 131.8, 127.7, 127.2, 117.5, 74.7( t ), 42.2, 38.6, 38.3, 26.8, 24.4. In vitro antifungal assays The MICs of the cationic compounds were measured using a broth microdilution method [22] . First, cationic compounds were dissolved in de-ionized (DI) water at 2,500 mg l −1 . The samples were further diluted to 31.25, 62.5, 125.0, 250.0, 500.0 and 1,000 mg l −1 . C. albicans and C. neoformans were grown in yeast mould broth (YMB) and Mueller Hinton broth (MHB), respectively, with vigorous shaking, and they were cultured at room temperature and 37 °C, respectively. The optical density (OD 600 nm ) of the fungus solution was adjusted to 0.1 by the addition of YMB or MHB. This fungus solution was further diluted to 10 5 CFU ml −1 using YMB or MHB. Cationic compound solution (100 μl) was transferred to each well of a 96-well plate (NUNC), followed by the addition of 100 μl of the fungus solution. YMB and MHB were used as the control. The optical density readings of fungus solutions were monitored by measuring OD 600 nm at predetermined times (0 h and 24 h) using a microplate reader (TECAN). The assay was performed in four replicates for each sample and the experiments were repeated at least three times. Antifungal activities of cationic compounds were further tested through a spread plate method. Briefly, C. albicans and C. neoformans were treated at specific concentrations of cationic compounds. At predetermined time points, microbial suspensions (20 or 100 μl) were withdrawn and diluted sequentially and then plated on 1.5% LB agar plates. The plates were incubated for 48 h at room temperature. Microbial colonies were formed and counted. The results were expressed as mean log 10 (CFU ml −1 ). The experiments were performed in triplicates, and were repeated three times. Drug resistance studies C. albicans was used as a model microbe for drug resistance studies. Drug resistance was induced by treating the C. albicans repeatedly with antimicrobial agents [23] . The MIC of 3b against C. albicans was tested for 11 passages of growth. MIC was determined using the broth microdilution method . C. albicans exposed to the sub-MIC concentration (1/8 of MIC at that particular passage) were re-grown to a logarithmic growth phrase, and re-used for the subsequent passage’s MIC measurement for the same antimicrobial agent. Drug-resistant behaviour of C. albicans was evaluated by recording the changes in the MIC normalized to that of the first passage. Conventional antifungal agent fluconazole was used as the control. Haemolysis assay Fresh rat blood cells were diluted with PBS buffer to give a cell suspension (4% in volume). Cell suspension (100 μl) was introduced to each well of a 96-well plate, and 100 μl of cationic compound solution was then added to the well. PBS and Triton X-100 (0.2%) were used as the control. The plates were incubated for 1 h at 37 °C. The 96-well plates were centrifuged at 2,200 r.p.m. for 5 min. Aliquots (100 μl) of the supernatant were transferred to a new 96-well plate. Haemoglobin release was measured at 576 nm using a microplate reader (TECAN). The red blood cells in PBS were used as a negative control. Absorbance of wells with red blood cells lysed with 0.2% Triton X-100 was taken as 100% haemolysis. Percentage of haemolysis was calculated using the following formula: haemolysis (%)=[(OD 576nm in the sample−OD 576nm in PBS)/(OD 576nm in 0.2% Triton X-100−OD 576nm in PBS)] × 100. The data were expressed as mean and s.d. of four replicates, and the tests were repeated three times. MTT assay The cytotoxicity tests of cationic compounds were performed in human dermal fibroblasts using MTT assay. The cells were cultured in Dulbecco’s Modified Eagle Medium (DMEM) supplemented with 10% FBS, 5% penicillin, 2 mM L -glutamine (Sigma) and incubated at 37 °C in 5% CO 2 . The cells were seeded onto 96-well plates at a density of 10,000 cells per well and incubated for 1 day. Cationic compounds were diluted with the growth medium to give final concentrations of 31.25, 62.50, 125.0, 250.0, 500.0 and 1,000 mg l −1 . The media were replaced with 100 μl of the pre-prepared samples. The plates were then returned to the incubator and maintained in 5% CO 2 at 37 °C for 24 h. Fresh growth media (100 μl) containing 10% MTT solution (5 mg ml −1 ) were used to replace the mixture in each well after 24 h. The plates were then returned to the incubator, and maintained in 5% CO 2 at 37 °C for another 4 h. The growth medium and excess MTT in each well were then removed. DMSO (150 μl) was then added to each well to dissolve the internalized purple formazan crystals. An aliquot of 100 μl was taken from each well, and transferred to a new 96-well plate. Each sample was tested in eight replicates per plate. The plates were then assayed at 550 nm and 690 nm. The absorbance readings of the formazan crystals were taken to be that at 550 nm subtracted by that at 690 nm. The results were expressed as a percentage of the absorbance of the blank control. SEM analysis The C. albicans before and after incubation with cationic compound 3b at MIC for 2 h were harvested by centrifugation at 4,000 r.p.m. for 5 min. They were washed by PBS three times, and then fixed in formalin solution containing 4% formaldehyde overnight. The cells were further washed with DI water, followed by dehydration using a series of ethanol solutions with different volume contents (35, 50, 75, 90, 95 and 100%). The sample was placed on a carbon tape, which was further coated with platinum. The morphologies of the C. albicans before and after the treatment were observed using a field emission scanning electron microscope (JEOL JSM-7400F) operated at an accelerating voltage of 10.0 kV and a working distance of 8.0 mm. TEM analysis The morphologies of the cationic compounds were analysed by TEM (FEI Tecnai G 2 F20 electron microscope). Samples were prepared by a membrane dialysis method. The cationic compounds (10 mg) were dissolved in 2 ml of DMF. The solution was then dialyzed against DI water at 20 °C for 24 h using a dialysis membrane with a molecular weight cutoff of 1,000 (Spectra/Por 7, Spectrum Laboratories Inc.). Cationic compounds solution (5 μl) was placed on a copper grid coated with carbon film and incubated for 1 min. Phosphotungstic acid (5 μl; 0.1 w/v%) was applied and incubated for another minute. The extra sample solution on the grid was absorbed by filter paper. The samples were air-dried at room temperature. The TEM studies were conducted with an electron kinetic energy of 200 keV. The morphologies of the C. neoformans before and after treatment with cationic compound 3b were observed under a JEM-1230 transmission electron microscope (JEOL, Japan) using an acceleration voltage of 80 keV. The C. neoformans (1.5 ml) were incubated with 0.5 ml of 3b solution at 2 × MIC for 8 h. The solution was then centrifuged at 4,000 r.p.m. for 10 min, and the supernatants were removed. They were washed by PBS (pH 7.0) twice, and then fixed in formalin solution containing 2.5% glutaraldehyde overnight. The samples were then washed by PBS three times (15 min each), and post-fixed with 1% OsO 4 in the phosphate buffer (pH 7.0) for 1 h. The fixed samples were washed in the phosphate buffer three times (15 min each), followed by dehydration in a graded ethanol solution series. The samples were incubated with a mixture of acetone and Spurr resin (1:1 in volume) for 1 h at room temperature, and then transferred to a 1:3 mixture of acetone and Spurr resin for 3 h, and lastly to Spurr resin for overnight incubation. Ultrathin sections (70–90 nm) were obtained with a Reichert–Jung Ultracut E ultramicrotome, and post-stained with uranyl acetate and lead citrate for 15 min each prior to the TEM studies. Membrane integrity test To further elucidate that the fungal membrane was damaged after the treatment, the presence of 260 nm-absorbing molecules in the culture media was tested after 3 h of incubation with the nanostructures according to a previously reported protocol [18] . Briefly, overnight culture of C. albicans was first adjusted to contain 3 × 10 6 CFU ml −1 with sterile PBS. Antifungal solutions were prepared at different concentrations of 3b by serial dilutions with sterile DI water. Equal volumes of fungal suspension and antifungal solution were then mixed to achieve the final 3b concentrations ranging from MIC to 4 × MIC, and the mixture was incubated for 3 h. The microbial suspension was filtered with 0.22-mm filter to remove the fungal cells from the suspension, and the absorbance of the filtrate solution was measured at 260 nm using a ultraviolet-visible spectrophotometer (Nanodrop ND-1000, Biofrontiers Technology, Singapore). The experiment was performed in triplicate, and untreated fungal suspension was used as the negative control to normalize the absorbance reading of the experimental groups. Biofilm formation C. albicans biofilm was formed on contact lenses (Air optix, CIBA Vision). The contact lens was cut into pieces of 2 mm in diameter and transferred into a six-well plate. The samples were soaked in YMB overnight at 37 °C. Broth solution was withdrawn from the plates, followed by addition of 4 ml of C. albicans (10 7 CFU ml −1 ) to each well. The plates were incubated at room temperature with shaking at 100 r.p.m. After 5 h of incubation, suspension was withdrawn and the lenses were washed by phosphate buffered saline (PBS) (pH 7.4) to remove any non-adherent cells, followed by the addition of 4 ml of fresh YMB. The plates containing the contact lenses with cells adhered were incubated at room temperature with shaking at 100 r.p.m. for 2 days to allow biofilm formation. In vitro anti-biofilm assays Contact lenses containing biofilms were transferred to individual wells of a new 24-well plate. Biofilms were washed three times using PBS (pH 7.4) to remove non-adhered cells. Solution (500 μl) containing different concentrations of 3b was added to each well containing biofilm, which was incubated for another day. Blank contact lenses were used as the control. After treatment, the solution was withdrawn from each well, and the biofilm was washed with PBS. The viability of cells in the biofilm was determined by XTT assay. This assay is based on the reduction of XTT tetrazolium salt to XTT formazan by mitochondrial dehydrogenases. Briefly, 200 μl of PBS containing 20 μl of XTT solution (1 mg ml −1 ) and 4 μl of menadione solution (1 mM) were added to each well. Plates were then incubated at 37 °C for 3 h. The colorimetric change associated with cell viability was measured using the microplate reader at 490 nm. The results were expressed as a percentage of the absorbance of the untreated samples. The ECM production was quantified by Safranin assay. Briefly, the biofilms were stained with 200 μl of aqueous solution containing 0.1% Safranin O for 15 min. The excess stain was removed by washing with PBS. The stained biofilm was solubilized with 200 μl of 70% ethanol for 15 min and the optical absorbance at 550 nm was recorded using the microplate reader. The assay was performed in four replicates for each sample, and the experiments were repeated at least three times. The readings were normalized to that of the untreated samples. The biofilm samples before and after 3b treatment (500 mg l −1 ) for SEM images were prepared using a similar method as described earlier. The biofilms formed on contact lenses were also observed with confocal laser scanning fluorescence microscopy (CLSM). Briefly, contact lenses containing biofilms before and after 3b treatment at 500 mg l −1 were washed three times using PBS, and transferred to individual wells of a new 24-well plate. The samples were stained with 1 ml of PBS solution containing 25 mg l −1 of green fluorescence CON-A (excitation wavelength: 488 nm; emission wavelength: 505 nm) and 10 μM of red fluorescence FUN-1 (excitation wavelength: 543 nm; emission wavelength: 560 nm) for 30 min at 37 °C, followed by rinsing with PBS solution. Samples were visualized by Carl Zeiss LSM 510 META confocal microscope (Germany). Three-dimensional (3D) reconstruction of images was obtained with Imaris software. All images were obtained under the same conditions. In vivo toxicity evaluation C57BL/6 mice (8 weeks old, 18–22 g) were used for animal studies. The mice were randomly grouped. In each group, a total of three mice were used. The compound 3b (2,000 mg l −1 in aqueous solution) was administered to the eyes every 5 min during the first hour and every 30 min during the next 7 h. All mice were killed after the administration of the last eye drop. The treated eyeballs were collected and fixed in 4% neutral buffered formalin. The fixed eyeballs were embedded in paraffin, sectioned and stained with hematoxylin (nucleus, blue) and eosin (cytoplasma, purple) by the standard protocol. The eyeballs treated with water were used as control. Keratitis model Keratitis model was established by a previously reported method [19] , [20] . The mice were immune suppressed via subcutaneously injecting cyclophosphamide (Sigma-Aldrich, 180 g per kg) at 5 days, 3 days and 1 day before inducing keratitis. The mice were anaesthetized by ketamine (150 mg per kg) and xylazine (10 mg ml −1 ) by intraperitoneal injection. Additional corneal anaesthesia was also performed with 0.5% tetracaine hydrochloride eye drops (Bausch & Lomb, Tampa, Florida). A 2-mm filter paper disc moistened with 99% 1-heptanol (Sigma-Aldrich, Lausanne, Switzerland) was placed on the centre of the cornea for 40 s. The corneal epithelium was wiped off and the eyes were rinsed with PBS removing any remaining 1-heptanol. A 2 mm-diameter punch from the contact lens with C. albicans biofilm was then placed on the denuded cornea surface. The lids were closed with silk sutures to keep the contact lenses inside. Eye ulcer with a leathery, tough and raised surface was observed after C. albicans were introduced on the eyeball for 18 h. The eye lids were then opened and the lens was removed. The mice with keratitis were randomly grouped in groups of nine and treated with three topical eye drop solutions: water (control), 2,000 mg l −1 of 3b and 1,500 mg l −1 of amphotericin B (AmB, Sigma-Aldrich, Lausanne, Switzerland). AmB was used as positive control. Eye drops (20 μl each) were administered to the mice every 5 min during the first hour and every 30 min during the next 7 h. The severity of keratitis was graded in clinical scores ranging from 1 to 12 based on the scoring system reported by Wu et al. [20] to evaluate treatment efficacy. A disease grading of 1–4 was assigned to the area of opacity, density of opacity and surface regularity ( Supplementary Table S2 ). A total score of ≤5, 6–9 and >9 indicate mild, moderate and severe keratitis, respectively. All mice were killed after the administration of the last eye drop. The treated eyeballs were collected immediately; three eyeballs from each group were collected for histology, and the remaining six eyeballs were homogenized (Pro200 tissue homogenizer) for quantitative analysis of fungal counts. Briefly, aliquots of serial dilutions were plated in triplicate on agar plates, and the plates were incubated for 48 h at room temperature before the colonies were counted. The number of CFUs recovered was expressed as mean log 10 CFU per eye. The fixed eyeballs were embedded in paraffin, sectioned and stained with Grocott’s methenamine silver or periodic acid-Schiff reagent by the standard protocol for histological analysis. To determine the extent of hyphal invasion into corneal stroma, each stained section obtained from cornea was imaged using a light microscope (Olympus, Japan). Three representative images per group with a total of 150 points (50 points for each image) were analysed for the absolute deepest depth of corneal penetration at each point using AutoCAD software. Statistics analysis The data were expressed as mean±s.d. (s.d. is indicated by the error bars). Student’s t -test was used to determine significance among groups. A value of P <0.05 was considered to be significant. How to cite this article: Fukushima, K. et al. Supramolecular high-aspect ratio assemblies with strong antifungal activity. Nat. Commun. 4:2861 doi: 10.1038/ncomms3861 (2013).